MicroRNA29aregulates IL-33-mediated tissue remodelling in tendon disease MicroRNA (miRNA) has the potential for cross-regulation and functional integration of discrete biological processes during complex physiological events. Utilizing the common human condition tendinopathy as a model system to explore the cross-regulation of immediate inflammation and matrix synthesis by miRNA we observed that elevated IL-33 expression is a characteristic of early tendinopathy. Using in vitro tenocyte cultures and in vivo models of tendon damage, we demonstrate that such IL-33 expression plays a pivotal role in the transition from type 1 to type 3 collagen (Col3) synthesis and thus early tendon remodelling. Both IL-33 effector function, via its decoy receptor sST2, and Col3 synthesis are regulated by miRNA29a . Downregulation of miRNA29a in human tenocytes is sufficient to induce an increase in Col3 expression. These data provide a molecular mechanism of miRNA-mediated integration of the early pathophysiologic events that facilitate tissue remodelling in human tendon after injury. Dysregulated tissue repair and inflammation characterize many common musculoskeletal pathologies [1] , including tendon disorders. Tendinopathies represent a common precipitant for musculoskeletal consultation in primary care [2] , [3] and comprise 30–50% of all sports injuries [3] . Tendinopathy is characterized by altered collagen production from subtype 1 to 3 resulting in a decrease in tensile strength that can presage clinical tendon rupture [4] . Inflammatory mediators are considered crucial to the onset and perpetuation of tendinopathy [5] . Expression of various cytokines has been demonstrated in inflammatory cell lineages and tenocytes suggesting that both infiltrating and resident populations participate in pathology [6] , [7] , [8] , [9] . Mechanical properties of healing tendons in interleukin (IL)-6-deficient mice are inferior compared with normal controls [10] , while tumour necrosis factor-α blockade improves the strength of tendon–bone healing in a rat tendon injury model [11] . While these data raise the intriguing possibility that cytokine targeting could offer therapeutic utility, there is currently insufficient mechanistic understanding of cytokine/matrix biology in tendon diseases to manifest this possibility in practice. IL-33 is a member of the IL-1 cytokine family that plays a major role in innate and acquired immune responses. IL-33 is expressed in endothelial cells and fibroblasts, co-located with chromatin in the nucleus [12] . IL-33 is released following cellular damage [13] and biomechanical overload [14] , and is thus considered an ‘alarmin’ [15] . It has been implicated in a variety of inflammatory pathologies including pulmonary, cutaneous and articular diseases [16] . IL-33 functions via its cognate receptor ST2 that exists in membrane-bound (mST2) or soluble decoy form (sST2) and signals via a canonical IL-1R signalling cascade. Cytokines are often regulated at the post-transcriptional level by miRNA that control the gene expression by translational suppression and destabilization of target mRNAs [17] . miRNA networks are emerging as key homeostatic regulators of tissue repair with fundamental roles proposed in stem cell biology, inflammation, hypoxia response and angiogenesis [18] . On the basis of the emerging role of fibroblast-derived IL-33 in inflammatory [19] , [20] and fibrotic disorders [21] and previous investigations showing increased inflammatory leukocyte infiltration in torn rotator cuff tendons [22] , we hypothesized that the IL-33/ST2 signalling pathway might play a significant role in tendon pathology. Our data derived in animal and human models of tendinopathy collectively suggest that the IL-33/ST2 system functions as an alarmin in tendon by triggering inflammation and switching collagen production towards biomechanically inferior collagen III synthesis, thus contributing to the severity of tendinopathy. Importantly, we found that miR-29a acts as a critical regulator of tenocyte biology by integrating IL-33 effector function and collagen matrix changes. This provides a novel insight into the coordinated regulation of disparate biochemical pathways by an miRNA to thereby modulate emerging tissue pathology. IL-33 and ST2 expression in human tendinopathy We first investigated IL-33 expression in human tendinopathy using our previously developed model [23] . IL33 , soluble and membrane-bound ST2 transcripts were significantly upregulated in early tendinopathy compared with control or torn tendon biopsies ( Fig. 1a–c ). Early tendinopathy tissues exhibited significantly greater staining for IL-33 and ST2 compared with torn tendon or control biopsies ( Fig. 1d ). Staining was prominent in endothelial cells (CD34 + ) and particularly fibroblast-like cells, namely tenocytes, which are considered pivotal to the regulation of early tendinopathy ( Supplementary Fig. 1a,b ). In parallel, in vitro -cultured tenocytes expressed nuclear IL-33 that was upregulated at both the mRNA and protein levels following stimulation by TNF-α and IL-1β ( Fig. 1e,f ). In contrast, ST2 was constitutively expressed in both resting and unstimulated tenocytes ( Supplementary Fig. 1c ). 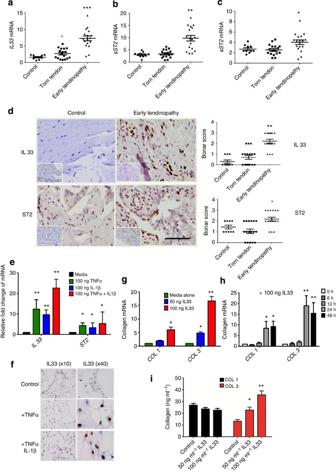Figure 1: IL-33/ST2 expression in human tendon. (a)IL-33, (b) soluble ST2 (sST2) and (c)mST2mRNA expression in human tendon samples. Fold change in gene expression of IL-33, sST2 and mST2 in control (semi-membranosus tendon,n=10), torn supraspinatus tendon (established pathology) and matched subscapularis human tendon samples (early pathology;n=17). Data are mean±s.d. relative to the housekeeping gene18S (mean of duplicate analysis). *P<0.05, **P<0.01, ***P<0.001 versus control (Student’st-test). (d) Immunostaining of IL-33 and ST2 in control (n=10), torn tendon (n=17) and early tendinopathy (n=17). Graphs illustrate modified Bonar scoring based on 10 high-power fields. Data are mean±s.d. *P<0.05, **P<0.01 versus control (Student’st-test). Scale bar, 65 μm. (e) Fold change in gene expression ofIL33andST224 h post incubation with tumour necrosis factor (TNF-α), IL-1β or in combination depicting relative expression to media alone utilizing housekeeping geneGAPDH. Data are mean±s.d. of triplicate samples, representative of three individual patient samples. *P<0.05, **P<0.01 versus control (media) (Student’st-test). (f) IL-33 immunostaining of human tendon explants cultured for 24 h with medium (control), 100 ng ml−1TNFα or 100 ng ml−1TNFα+100 ng ml−1IL-1β. (g) Fold change inCOL1andCOL3mRNA expression in human tendon explants cultured for 24 h with rhIL-33, relative to housekeeping geneGAPDH. (h) Time course ofCOL1andCOL3mRNA expression following incubation with rhIL-33, relative to housekeeping geneGAPDH. (i) Collagen 1 and 3 protein expression in human tendon explants 24 h post incubation with rhIL-33. For (g–i) data are mean±s.d. of triplicate samples, representative of three individual patients. *P<0.05, **P<0.01 versus control (Student’st-test). Figure 1: IL-33/ST2 expression in human tendon. ( a ) IL-33 , ( b ) soluble ST2 ( sST2 ) and ( c ) mST2 mRNA expression in human tendon samples. Fold change in gene expression of IL-33, sST2 and mST2 in control (semi-membranosus tendon, n =10), torn supraspinatus tendon (established pathology) and matched subscapularis human tendon samples (early pathology; n =17). Data are mean±s.d. relative to the housekeeping gene18S (mean of duplicate analysis). * P <0.05, ** P <0.01, *** P <0.001 versus control (Student’s t- test). ( d ) Immunostaining of IL-33 and ST2 in control ( n =10), torn tendon ( n =17) and early tendinopathy ( n =17). Graphs illustrate modified Bonar scoring based on 10 high-power fields. Data are mean±s.d. * P <0.05, ** P <0.01 versus control (Student’s t -test). Scale bar, 65 μm. ( e ) Fold change in gene expression of IL33 and ST2 24 h post incubation with tumour necrosis factor (TNF-α), IL-1β or in combination depicting relative expression to media alone utilizing housekeeping gene GAPDH . Data are mean±s.d. of triplicate samples, representative of three individual patient samples. * P <0.05, ** P <0.01 versus control (media) (Student’s t -test). ( f ) IL-33 immunostaining of human tendon explants cultured for 24 h with medium (control), 100 ng ml −1 TNFα or 100 ng ml −1 TNFα+100 ng ml −1 IL-1β. ( g ) Fold change in COL1 and COL3 mRNA expression in human tendon explants cultured for 24 h with rhIL-33, relative to housekeeping gene GAPDH . ( h ) Time course of COL1 and COL3 mRNA expression following incubation with rhIL-33, relative to housekeeping gene GAPDH . ( i ) Collagen 1 and 3 protein expression in human tendon explants 24 h post incubation with rhIL-33. For ( g – i ) data are mean±s.d. of triplicate samples, representative of three individual patients. * P <0.05, ** P <0.01 versus control (Student’s t -test). Full size image IL-33 regulates tenocyte collagen matrix and cytokine synthesis Matrix dysregulation towards collagen 3 (Col3) expression is a key early phenotypic change in tendinopathy thereby hastening repair; Col3 is however biomechanically inferior [4] . IL-33 induced dose- and time-dependent upregulation of total collagen protein ( Supplementary Fig. 1d ), accounted for by an increased expression of type I but particularly type III collagen mRNA and protein ( Fig. 1g–i , Supplementary Fig. 1e ). Following array analysis ( Supplementary Fig. 2a–c ) and consistent with reported IL-33 downstream signalling [12] , [16] . IL-33-induced collagen expression was abrogated by ERK and NFκB inhibition ( Supplementary Fig. 2d,e ). Recombinant IL-33 also significantly elevated the production of IL-6, IL-8 and monocyte chemoattractant protein-1, which was abrogated by NF-κB inhibition ( Supplementary Fig. 2f ), suggesting that IL-33 operates in tenocytes via its canonical IL-1R signalling pathway. Modelling IL-33/ST2 pathway in vivo following tendon injury We extended these observations to a well-established in vivo murine model of tendon injury. IL-33 mRNA and protein were elevated on days 1 and 3 post tendon injury in wild-type (WT) BALB/c mice ( Fig. 2a–c ). This was significantly reduced in injured St2 −/− BALB/c mice suggesting autocrine regulation. Soluble St2 was significantly upregulated at all time points post injury in WT mice compared with uninjured controls ( Fig. 2b ). No significant changes in Il33 or St2 transcript were found in WT mice at days 7 or 21 post injury, or for Il33 expression in St2 −/− mice, suggesting that the impact of IL-33 expression is manifest early, in keeping with ‘alarmin’ type activity in tendon injury/repair. 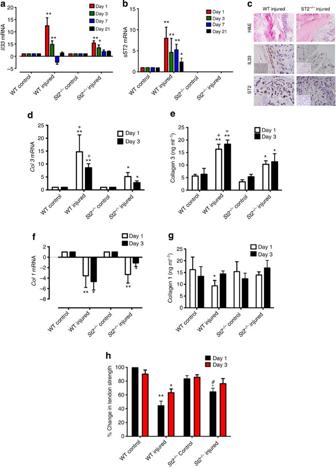Figure 2: IL-33/ST2 axis in tendon healingin vivo. Kinetics of (a)Il33and (b) solubleSt2gene expression post injury. Data are mean fold change±s.d. showing relative expression to18shousekeeping gene (pooled data from four mice per group performed on four sequential occasions,n=16 per condition). *P<0.05, **P<0.01 versus control (WT) mice (ANOVA) +P<0.05,++P<0.01, NS not significant; control (WT) injured versusSt2−/−injured. (c) Immunohistochemistry showing IL-33 and ST2 expression in tendon biopsies of WT andSt2−/−mice day 1 post injury. IgG control shown in bottom left of pictures. Black horizontal line indicates 50 μm. (d)Col3mRNA and (e) Collagen 3 protein levels in tendon biopsies of WT andSt2−/−mice post injury. (f)Col1mRNA and (g) Collagen 1 protein levels in tendon biopsies of WT andSt2−/−mice post injury. For (d–g) data are mean±s.d. of duplicate samples, representative of four mice per condition (n=16). *P<0.05, **P<0.01 versus control (WT) mice. +P<0.05, ++P<0.01 control (WT) injured versusSt2−/−injured mice (ANOVA). mRNA graphs show relative expression to18shousekeeping gene. (h) Percentage change in tendon strength for WT andSt2−/−mice post injury. Data are mean±s.d., representative of four mice per condition (n=16). *P<0.05, **P<0.01 versus control mice.#P<0.05St2−/−injured versus WT injured mice (Mann–WhitneyU-test). Figure 2: IL-33/ST2 axis in tendon healing in vivo . Kinetics of ( a ) Il33 and ( b ) soluble St2 gene expression post injury. Data are mean fold change±s.d. showing relative expression to 18s housekeeping gene (pooled data from four mice per group performed on four sequential occasions, n =16 per condition). * P <0.05, ** P <0.01 versus control (WT) mice (ANOVA) + P <0.05,++ P <0.01, NS not significant; control (WT) injured versus St2 −/− injured. ( c ) Immunohistochemistry showing IL-33 and ST2 expression in tendon biopsies of WT and St2 −/− mice day 1 post injury. IgG control shown in bottom left of pictures. Black horizontal line indicates 50 μm. ( d ) Col3 mRNA and ( e ) Collagen 3 protein levels in tendon biopsies of WT and St2 −/− mice post injury. ( f ) Col1 mRNA and ( g ) Collagen 1 protein levels in tendon biopsies of WT and St2 −/− mice post injury. For ( d – g ) data are mean±s.d. of duplicate samples, representative of four mice per condition ( n =16). * P <0.05, ** P <0.01 versus control (WT) mice. + P <0.05, ++ P <0.01 control (WT) injured versus St2 −/− injured mice (ANOVA). mRNA graphs show relative expression to 18s housekeeping gene. ( h ) Percentage change in tendon strength for WT and St2 −/− mice post injury. Data are mean±s.d., representative of four mice per condition ( n =16). * P <0.05, ** P <0.01 versus control mice. # P <0.05 St2 −/− injured versus WT injured mice (Mann–Whitney U -test). Full size image Analysis of collagen synthesis revealed significantly greater expression of collagen 3 at all time points post injury in WT mice compared with uninjured controls or injured St2 −/− mice ( Fig. 2d,e and Supplementary Fig. 3 ). Collagen 1 was initially downregulated (days 1, 3) at mRNA levels ( Fig. 2f ) in injured WT mice but reverted towards pre-injury levels by days 7 and 21 ( Supplementary Fig. 3a ) with a similar trend in Collagen 1 protein expression ( Fig. 2g ). In contrast, injured St2 −/− mice showed prolonged reduction of collagen 1 synthesis (days 1, 3 and 7) returning to baseline only by day 21 ( Supplementary Fig. 3d ). Importantly, injury of WT mice tendons resulted in a significant decrease in biomechanical strength at day 1 post injury compared with that of the St2 −/− mice ( Fig. 2h ). The biomechanical strength in all injured mice recovered by days 7 and 21 ( Supplementary Fig. 3f ). These data suggest altered collagen matrix synthesis in St2 −/− mice implicating IL-33/ST2 as an early modulator of collagen changes in tendon injury that has biomechanical significance. IL-33 modifies collagen 3 expression in vivo To confirm that IL-33 regulates collagen synthesis during tendon injury, we sought to directly modify IL-33 effector function in vivo . Administration of rhIL-33 did not affect collagen 1 synthesis ( Fig. 3a,b ), but significantly increased collagen 3 synthesis particularly in injured tendons ( Fig. 3c,d and Supplementary Fig. 4a,b ). Moreover, rhIL33 administration significantly reduced ultimate tendon strength at all time points post injection in WT mice ( Fig. 3e and Supplementary Fig. 4c,d ) suggesting that such changes were of functional impact. IL-33 administration did not affect collagen matrix synthesis or ultimate tendon strength of the healing tendon in St2 −/− mice confirming that IL-33 acted via an ST2-dependent pathway ( Supplementary Fig. 4 ). 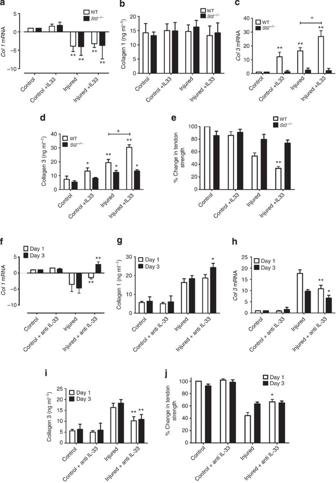Figure 3: IL-33/anti-IL-33 effects on collagen production and tendon strengthin vivo. (a)Col1mRNA, (b) Collagen 1 protein, (c)Col3mRNA and (d) Collagen 3 protein in WT andSt2−/−mice on day 1 post injury. mRNA graphs show relative expression to18shousekeeping gene. Data are mean±s.d. of duplicate samples, representative of four mice per condition (n=16). *P<0.05,**P<0.01, injured versus uninjured mice.+P<0.05 WT versus ST2−/−mice. (ANOVA). (e) Percentage change in tendon strength in WT and St2−/−mice on day 1 post injury with or without rhIL-33 treatment. Data are mean±s.d., representative of four mice per group (n=16). **P<0.01, injured versus injured+IL-33 mice (Mann–WhitneyU-test). (f)Col1mRNA, (g) Collagen 1 protein, (h)Col3mRNA, (i) Collagen 3 protein levels and (j) percentage change in tendon strength post tendon injury in WT mice with or without anti-IL-33 treatment. Data for mRNA show relative expression to18shousekeeping gene. Data are mean±s.d., representative of four mice per condition (n=16). *P<0.05, **P<0.01, injured versus uninjured mice (Mann–WhitneyU-test). Figure 3: IL-33/anti-IL-33 effects on collagen production and tendon strength in vivo . ( a ) Col1 mRNA, ( b ) Collagen 1 protein, ( c ) Col3 mRNA and ( d ) Collagen 3 protein in WT and St2 −/− mice on day 1 post injury. mRNA graphs show relative expression to 18s housekeeping gene. Data are mean±s.d. of duplicate samples, representative of four mice per condition ( n =16). * P <0.05,** P <0.01, injured versus uninjured mice. + P <0.05 WT versus ST2 −/− mice. (ANOVA). ( e ) Percentage change in tendon strength in WT and St2 −/− mice on day 1 post injury with or without rhIL-33 treatment. Data are mean±s.d., representative of four mice per group ( n =16). ** P <0.01, injured versus injured+IL-33 mice (Mann–Whitney U -test). ( f ) Col1 mRNA, ( g ) Collagen 1 protein, ( h ) Col3 mRNA, ( i ) Collagen 3 protein levels and ( j ) percentage change in tendon strength post tendon injury in WT mice with or without anti-IL-33 treatment. Data for mRNA show relative expression to 18s housekeeping gene. Data are mean±s.d., representative of four mice per condition ( n =16). * P <0.05, ** P <0.01, injured versus uninjured mice (Mann–Whitney U -test). Full size image We next directly targeted IL-33 in vivo . Neutralizing antibodies to IL-33 attenuated the collagen 1 to 3 switch at days 1 and 3 post injury in injured WT mice ( Fig. 3f–i , Supplementary Fig. 5a ) resulting in a significant increase in biomechanical strength at day 1 post injury in the tendons of WT mice ( Fig. 3j ). This effect was not seen at later time points ( Supplementary Fig. 5b ). In control experiments, we observed no effect of rIL-33 on St2 −/− mice ( Supplementary Fig. 5c,d ). These results, therefore, further demonstrate the contribution of endogenous IL-33 to early injury-induced tendinopathy. IL33 regulates collagen 3 via miR-29a in tenocytes Having established that IL-33 drives the differential regulation of collagen 1 and 3 in tenocytes, we postulated a mechanistic role for the miRNA network in this process. Previous studies have shown that the miR-29 family directly targets numerous extracellular matrix genes, including type 1 and 3 collagens [24] , [25] and is implicated in the regulation of innate and adaptive immunity [26] . Computational algorithms predict that miR-29 may also target sST2 (ref. 27 ). We found that all members of the miR-29 family were expressed in human tendon biopsies and explanted tenocytes ( Fig. 4a ) with miR-29a showing the most altered expression in early tendinopathy biopsies. In tenocyte culture, IL-33 significantly reduced the expression of miR-29a at 6, 12 and 24 h ( Fig. 4b ), whereas the effect on miR-29b was modest and highly variable ( Supplementary Fig. 6a ). The effect of IL-33 on miR-29a expression was NF-κB dependent ( Supplementary Fig. 6b ). Since IL-33-mediated collagen 3 matrix changes could be regulated by miR-29a , we analysed the functional effects of miR-29a manipulation on collagen matrix synthesis in vitro . Using luciferase assays, we first confirmed that miR-29a directly targets COL 1A1 and 3A1 as previously demonstrated [28] ( Supplementary Fig. 6c ). We also observed a previously unrecognized interaction of miR-29a with human COL 1A2 subunit transcript ( Fig. 4c ). To test whether miR-29a indeed regulates the levels of candidate target mRNAs in disease relevant cells, we transfected tenocytes with miR-29a mimic and antagomir. miR-29a manipulation selectively regulated collagen 3 but not collagen 1 mRNA and protein expression in primary tenocytes ( Fig. 4d,e ). Moreover, miR-29a overexpression significantly decreased IL-33-induced collagen 3 mRNA and protein synthesis ( Supplementary Fig. 6d and Fig. 4f ). In additiona, miR-29a inhibition resulted in a significant increase in COL 3A1 expression ( Fig. 4g ), indicating that miR-29a is not only actively regulating these transcripts in human tenocytes but its loss can be an important factor in the increase of type 3 collagen production observed in tendinopathy. In contrast, COL 1A1 and A2 transcript levels were relatively unchanged ( Fig. 4g ). 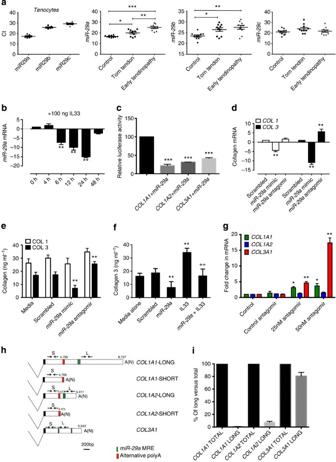Figure 4: IL33 promotes differential regulation of collagen 1 and 3 viamiR-29ain human tenocytes. (a) Expression (Ct, threshold cycle values; lowerCt=more abundance expression) ofmiR-29a,miR-29bandmiR-29cin tenocytes (n=6) and relative fold change toU6housekeeping in control, torn supraspinatus (torn tendon) and matched subscapularis tendon (early tendinopathy). Data are mean±s.d. of duplicate samples and represent experiments on 10 patient samples. *P<0.05, **P<0.01. (Student’st-test). (b) Time course ofmiR-29aexpression in human tenocytes following cultured with rhIL-33 showing relative fold change toU6housekeeping. (c) Luciferase activity in primary human tenocytes transfected with precursormiR-29acontaining 3′UTR ofCOL1A1,COL1A2orCOL3A1. Activity was determined relative to controls transfected with scrambled RNA, which was defined as 100%. This was repeated in three independent experiments. **P<0.01, **P<0.01 versus scrambled control. (Student’st-test). (d)COL1andCOL3mRNA and (e) collagen 1 and 3 protein expression following transfection with scrambled mimic,miR-29amimic ormiR-29aantagomir. (f) Collagen 3 protein levels following addition ofmiR-29amimic/antagomir and 100 ng rhIL-33. Forc–f, data shown are mean±s.d. of duplicate samples and represent experiments on five tendon explant samples, (n=5). *P<0.05, **P<0.01 versus scrambled control,++P<0.01 versus withoutmiR-29a. (ANOVA). (g)COL1A1,COL1A2andCOL3A1mRNA in human tenocytes following transfection with scrambled mimic (control antagomir) ormiR-29aantagomir showing relative fold change toU6housekeeping. Data are mean±s.d. of duplicate samples and represent experiments on three tendon explant samples. (n=3). *P<0.05, **P<0.01 versus control (Mann–WhitneyU-test). (h) Schematic diagram of alternative polyadenylated 3′UTRs fromCOL1A1,COL1A2 and COL3A1, showing the positions ofmiR-29a-binding sites, qPCR primers and polyadenylation signals. A (N), polyadenylation. (i) Relative contribution of the long 3′UTR forms ofCOL1A1,COL1A2andCOL3A1to their total transcript levels was measured by qPCR (location of primers shown inh,n=3). Figure 4: IL33 promotes differential regulation of collagen 1 and 3 via miR-29a in human tenocytes. ( a ) Expression ( C t, threshold cycle values; lower C t=more abundance expression) of miR-29a , miR-29b and miR-29c in tenocytes ( n =6) and relative fold change to U6 housekeeping in control, torn supraspinatus (torn tendon) and matched subscapularis tendon (early tendinopathy). Data are mean±s.d. of duplicate samples and represent experiments on 10 patient samples. * P <0.05, ** P <0.01. (Student’s t -test). ( b ) Time course of miR-29a expression in human tenocytes following cultured with rhIL-33 showing relative fold change to U6 housekeeping. ( c ) Luciferase activity in primary human tenocytes transfected with precursor miR-29a containing 3′UTR of COL1A1 , COL1A2 or COL3A1 . Activity was determined relative to controls transfected with scrambled RNA, which was defined as 100%. This was repeated in three independent experiments. ** P <0.01, ** P <0.01 versus scrambled control. (Student’s t -test). ( d ) COL1 and COL3 mRNA and ( e ) collagen 1 and 3 protein expression following transfection with scrambled mimic, miR-29a mimic or miR-29a antagomir. ( f ) Collagen 3 protein levels following addition of miR-29a mimic/antagomir and 100 ng rhIL-33. For c – f , data shown are mean±s.d. of duplicate samples and represent experiments on five tendon explant samples, ( n =5). * P <0.05, ** P <0.01 versus scrambled control, ++ P<0.01 versus without miR-29a . (ANOVA). ( g ) COL1A1 , COL1A2 and COL3A1 mRNA in human tenocytes following transfection with scrambled mimic (control antagomir) or miR-29a antagomir showing relative fold change to U6 housekeeping. Data are mean±s.d. of duplicate samples and represent experiments on three tendon explant samples. ( n =3). * P <0.05, ** P <0.01 versus control (Mann–Whitney U -test). ( h ) Schematic diagram of alternative polyadenylated 3′UTRs from COL1A1 , COL1A2 and COL3A1 , showing the positions of miR-29a -binding sites, qPCR primers and polyadenylation signals. A (N), polyadenylation. ( i ) Relative contribution of the long 3′UTR forms of COL1A1 , COL1A2 and COL3A1 to their total transcript levels was measured by qPCR (location of primers shown in h , n =3). Full size image Given that miR-29a was capable of repressing COL 1A1 and 1A2 with equal or greater efficiency than collagen 3 in luciferase reporter assays, this was unlikely to be the result of miR-29a having greater affinity for its microRNA (miRNA) recognition element (MREs) in type 3 transcripts. One well-documented mechanism by which transcripts modulate their sensitivity to miRNA regulation is through the utilization of alternative polyadenylation signals ( Fig. 4h ) [29] . Use of distal polyadenylation signals results in reduction in 3′ untranslated region (UTR) length with the loss of MREs. To test this, we compared the levels of full-length ( miR-29a MRE containing) COL1A1 , COL1A2 and COL3A1 transcripts expressed in human tenocytes with their total levels by quantitative PCR (qPCR; Fig. 4i ). We found that 95% of COL1A1 and 1A2 transcripts did not contain miR-29a MRE, whereas the majority ( ∼ 75%) of COL3A1 transcripts did. 3′ rapid amplification of complementary DNA (cDNA ends, RACE; Supplementary Fig. 6e ) confirming that both COL1A1 and 1A2 make use of previously unrecognized polyadenylation signals ( Fig. 4h ). Analysis of COL3A1 3′RACE products identified transcripts containing a single miR-29a MRE due to use of a proximal polyadenylation signal. COL3A1 luciferase constructs, which contained only this MRE, were still efficiently repressed by miR-29a indicating that all COL3A1 transcripts are sensitive to regulation by miR-29a ( Supplementary Fig. 6f ). Inspection of 3′RACE sequences revealed the presence of canonical polyadenylation signals upstream of polyA tails. The resulting truncated COL1A1 and 1A2 3′UTRs lack miR-29a MREs. These data suggest that in tenocytes miR-29a specifically regulates COL3A1 , while both COL1A1 and COL1A2 are rendered insensitive to miR-29a inhibition due to the utilisation of alternative polyadenylation signals. Loss of miR-29a on IL-33 signalling results in the derepression of collagen 3 likely contributing to the increase of this collagen observed in injured tendons. Soluble ST2 is a direct target of miR-29a Computational analysis revealed that miR-22 , 183 , 25 and 29a were predicted to regulate sST2 . However, miR-22 , 183 and 25 showed much less favourable probability in targeting sST2 (total context score value [27] ) than miR-29 family. Importantly, only miR-29 family members showed a good probability in targeting both collagens and sST2 , thus suggesting a feasible regulatory role in IL-33 effector functions. A luciferase reporter gene was generated that contains the 3′UTR of human sST2 predicted to possess two potential miR-29abc -binding sites ( Supplementary Fig. 6g ). Co-transfection of sST2 -luciferase reporter plasmid with miR-29 mimics in HEK 293 cells resulted in significant reduction in luciferase activity relative to scrambled control ( Supplementary Fig. 6h ). Furthermore, luciferase activity was fully restored when the seed regions of both miR-29 MREs in sST2 were mutated, demonstrating that sST2 is a direct target of miR-29a ( Fig. 5a ). To investigate whether miR-29a does indeed regulate the levels of the candidate target mRNA in tenocytes, we again transfected miR-29a mimic or antagomir into human tenocytes. Soluble ST2 message was significantly decreased by transfection with miR-29a mimic and increased by antagomir ( Fig. 5b ), with a corresponding significant change in soluble ST2 protein ( Fig. 5c ). These results confirm soluble ST2 as a target of miR-29a . We also noted that miR-29a mimic transfection produced no effect on the production of rhIL-33-induced cytokines (IL-6, IL-8 and monocyte chemoattractant protein-1; Supplementary Fig. 6i ), suggesting that miR-29a is not directly involved in the regulation of IL-33 canonical IL-1R signalling in tenocytes. 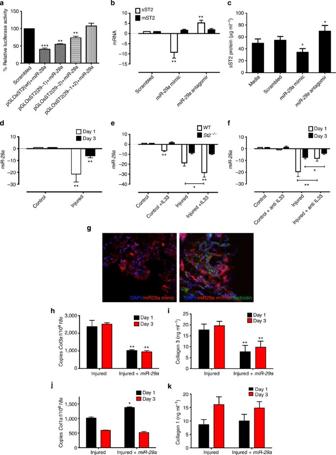Figure 5: Crosstalk between IL-33/ST2 andmiR-29a. (a) Luciferase activity assay of HEK 293 cells co-transferred with pre-miR-29acontaining 3′UTR of WT or mutated solubleST2and MREs of 3′UTR of solubleST2. (n=3). **P<0.01, ***P<0.001 versus scrambled control. (Student’st-test). (b)sST2andmST2mRNA levels following addition of scrambled mimic,miR-29amimic ormiR-29aantagomir in human tenocyte cultures. (n=5), **P<0.01 versus scrambled control (Student’st-test). (c) sST2 protein production by tenocytes following incubation withmiR-29amimic/antagomir. (n=5), *P<0.05 versus scrambled control. (Student’st-test). (d) qPCR showing fold change inmiR-29ain tendon of WT mice post injury. (e) qPCR showing fold change inmiR-29ain WT andSt2−/−mice following treatment with rhIL-33 or PBS on Day 1 post injury. (f)miR-29aexpression in the tendon of WT mice post injury with or without anti-IL-33 treatment. Data ind–fare mean fold change±s.d. of duplicate samples and are representative of four mice per group (n=16), *P<0.05, **P<0.01 versus control (ANOVA). Data for mRNA show expression relative tou6housekeeping gene. (g) Immunofluorescence stain of mimic (red) and counterstained with phalloidin (green, for cytoskeletal structure) showing localization of mimic around tenocytes at 24 h post injection of miR-29a mimic in WT mice. Scale bar, 80 nm. (h)Col3mRNA, (i) Collagen 3 protein, (j)Col1mRNA and (k) Collagen 1 protein levels post treatment withmiR-29amimic after tendon injury in WT mice. Data for mRNA are total copy number of gene versus 18S housekeeping gene in duplicate samples. Data inh–kare mean±s.d. of duplicate samples, representative of six mice per group, *P<0.05, **P<0.01 versus control (ANOVA). Figure 5: Crosstalk between IL-33/ST2 and miR-29a . ( a ) Luciferase activity assay of HEK 293 cells co-transferred with pre- miR-29a containing 3′UTR of WT or mutated soluble ST2 and MREs of 3′UTR of soluble ST2 . ( n =3). ** P <0.01, *** P <0.001 versus scrambled control. (Student’s t -test). ( b ) sST2 and mST2 mRNA levels following addition of scrambled mimic, miR-29a mimic or miR-29a antagomir in human tenocyte cultures. ( n =5), ** P <0.01 versus scrambled control (Student’s t -test). ( c ) sST2 protein production by tenocytes following incubation with miR-29a mimic/antagomir. ( n =5), * P <0.05 versus scrambled control. (Student’s t -test). ( d ) qPCR showing fold change in miR-29a in tendon of WT mice post injury. ( e ) qPCR showing fold change in miR-29a in WT and St2 −/− mice following treatment with rhIL-33 or PBS on Day 1 post injury. ( f ) miR-29a expression in the tendon of WT mice post injury with or without anti-IL-33 treatment. Data in d – f are mean fold change±s.d. of duplicate samples and are representative of four mice per group ( n =16), * P <0.05, ** P <0.01 versus control (ANOVA). Data for mRNA show expression relative to u6 housekeeping gene. ( g ) Immunofluorescence stain of mimic (red) and counterstained with phalloidin (green, for cytoskeletal structure) showing localization of mimic around tenocytes at 24 h post injection of miR-29a mimic in WT mice. Scale bar, 80 nm. ( h ) Col3 mRNA, ( i ) Collagen 3 protein, ( j ) Col1 mRNA and ( k ) Collagen 1 protein levels post treatment with miR-29a mimic after tendon injury in WT mice. Data for mRNA are total copy number of gene versus 18S housekeeping gene in duplicate samples. Data in h – k are mean±s.d. of duplicate samples, representative of six mice per group, * P <0.05, ** P <0.01 versus control (ANOVA). Full size image IL-33/sST2 regulates miR-29a expression in tendon healing We next investigated miR-29a expression in our in vivo tendon-healing model. Tendon injury in WT mice resulted in a 22-fold decrease in miR-29a on day 1, which reverted to a sixfold decrease (versus baseline) by day 3 ( Fig. 5d and Supplementary Fig. 7a ) with no significant difference by day 7. This effect was significantly decreased in St2 −/− mice ( Supplementary Fig. 7a ). In addition, the administration of exogenous rhIL-33 reduced miR-29a expression in uninjured tendons at all time points compared with PBS-injected controls ( Supplementary Fig. 7b ). This effect was most profound in injured WT mice, with the addition of rhIL-33 mediating a further 10-fold reduction in miR-29a ( Fig. 5e ). Addition of rhIL-33 in St2 −/− mice had no significant effect on miR-29a expression in injured or uninjured tendons ( Fig. 5e ), again suggesting that miR-29a downregulation is, at least in part, directly mediated by IL-33/ST2-dependent signalling. The addition of neutralizing antibody to IL-33 significantly reduced the effect of injury on miR-29a gene expression at days 1 and 3 post injury ( Fig. 5f ). Overexpression of miR-29a regulates collagen changes in vivo Finally, based on our observations that the reduction of miR-29a function was linked to collagen matrix changes in human and animal models of tendon disease, we investigated the role of overexpression of miR-29a in vivo in an attempt to reverse these changes. Delivery of miR-29a mimic to the in vivo tendon-healing model, with tissue uptake confirmed by immunofluorescence and qPCR ( Fig. 5g and Supplementary Fig. 7c ), resulted in a significant reduction ( P <0.01) of collagen 3 synthesis at days 1 and 3 post injury ( Fig. 5h,i ). While a transient increase in Col1 message was noted at day 1 post injury ( Fig. 5j ), miR-29a overexpression caused no reduction in collagen 1 protein levels in vivo at days 1 and 3 post injury compared with control samples ( Fig. 5k ). miRNAs have emerged as powerful regulators of diverse cellular processes with important roles in disease and tissue remodelling. Studies reported here using tendinopathy as a model system reveal the previously unrecognized ability of a single miRNA ( miR-29a ) to cross-regulate inflammatory cytokine effector function and extracellular matrix in the complex early biological processes leading to tissue repair. We also provide evidence for a hitherto unreported role of IL-33 in the initial steps that lead to the important clinical entity of tendinopathy. IL-33 has recently become increasingly associated with musculoskeletal pathologies [16] . Our data show IL-33 to be present in human tendon biopsies at the early stage of disease, while end-stage biopsies have significantly less IL-33 expression at the message and protein level supporting the concept of IL-33 as an early tissue mediator in tendon injury and subsequent tissue remodelling. On cell injury, the so-called alarmins such as heat shock proteins [30] , HMGB1 (ref. 31 ), uric acid [32] and IL-1 family members [33] , [34] , including IL-33 (refs 35 , 36 ), are released by both resident immune cells and necrotic cells having undergone damage. These alarmins are subsequently recognized by various immune cells that initiate inflammatory and repair responses. Our data implicate IL-33 as an alarmin in early tendinopathy and, importantly, our biomechanical data suggest that such an expression has a pathogenically relevant role. The addition of rhIL-33 significantly reduced the tendon strength (load to failure) of WT mice by ∼ 30% at early time points, likely as a consequence of the concomitant collagen 3 matrix changes, which result in mechanically inferior tendon [37] . Thus, one plausible mechanism for the events, mediating early biomechanically inferior tendon repair, is that on repeated micro injury IL-33 is upregulated with its subsequent release through mechanical stress/necrosis. IL-33 then drives the matrix degeneration and proinflammatory cytokine production, propelling the tendon towards a pathological state such as that seen in early tendinopathy biopsies. Interestingly, the addition of IL-33-neutralizing antibodies to injured mice reversed the collagen 3 synthesis, but this was only able to temporarily improve tendon strength on day 1 post injury. While this may negate blocking IL-33 in longer-term sports injuries, the repetitive microtrauma associated with pathological tendon changes may conversely allow neutralizing IL-33 to act as a check rein to further unwanted matrix dysregulation. Although these results do not exclude the contribution of other immune cells to IL-33-mediated tendon pathology, our in vitro studies performed on tenocytes show a robust effect of IL-33 on the differential collagen 1:3 ratio, which is replicated in the in vivo setting. Thus, while immune cells will undoubtedly be relevant to tendon damage in vivo, our results support the notion that tenocytes are of substantial significance in the IL-33-mediated changes in tendon injury. Emerging studies highlight miRNAs as key regulators of leukocyte function and the cytokine network while orchestrating proliferation and differentiation of stromal lineages that determine extracellular matrix composition [38] . The finding of a key role for miR-29a in the regulation of IL-33 ‘alarmin’-mediated effects provides mechanistic insight into miRNA cross-regulatory networks involving inflammation and matrix regulation in tissue repair. Our data demonstrate a functional role for miR-29a as a post-transcriptional regulator of collagen in murine and human tendon injury. The regulation of collagens and other extracellular matrices by the miR-29 family has been highlighted in several prior studies [28] , [29] , [39] , [40] , [41] . Our results now suggest that miR-29a acts as a critical repressor to regulate collagen expression in tendon healing. Moreover, the reduced expression of miR-29a in human biopsies suggests that its functional diminution leads to development of tendinopathy. Despite tendon pathology being characterized by increased collagen 3 deposition resulting in biomechanical inferiority and degeneration, the molecular premise for this collagen ‘switch’ has hitherto been unknown. We describe here that IL-33-induced deficiency in miR-29a results in an overproduction of collagen 3 while simultaneously setting in motion, via sST2 inhibition of IL-33, the ultimate resolution of this early repair process ( Fig. 6 ). Contrary to expectations in human tenocytes, miR-29a was only capable of influencing the expression of COL3A1 and not type 1 collagens. Subsequent characterization of the 3′UTR of type 1 and 3 collagens revealed a previously unreported pattern of alternative polyadenylation in both type 1 subunits, resulting in transcripts lacking miR-29a -binding sites rendering them insensitive to repression by this miRNA. This was not the case for type 3 collagen transcripts, which retain miR-29a -binding sites. In human tenocytes, collagen 3 is actively repressed by miR-29a , as demonstrated by the ability of miR-29a inhibitors to significant increase collagen 3 levels. Furthermore, supplementing tenocytes with miR-29a in the presence of IL-33 was sufficient to inhibit the increased production of collagen 3. These results indicate that miR-29a -mediated regulation of collagen 3 transcript stability is the predominant factor in the observed increased collagen 3 production. Importantly, in our model system, miR-29a additionally targeted the IL-33 decoy receptor sST2. Thus, IL-33-driven loss of miR-29a expression results in the simultaneous repression of collagen 3 and sST2, with a subsequent autoregulatory inhibition of IL-33 promoting the resolution of the immediate alarmin response. Alternative miRNAs have been described at various stages of the tendinopathy spectrum [42] , [43] . While it is likely that miR29a targets other important genes [44] , [45] in the complex tendon inflammatory/matrix mileu, our data suggest that the reintroduction of miR-29a to the injury-induced miR-29a deficiency in tendon results in reversal of the key collagen switch that remains a core pathological feature of tendinopathy linked to ultimate clinical tendon rupture. 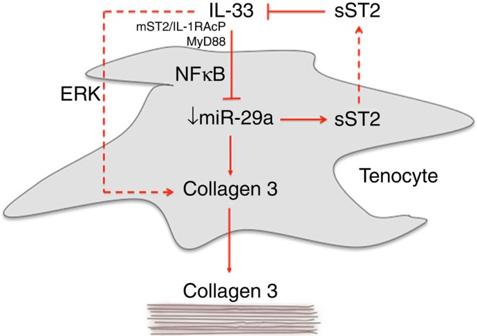Figure 6: Schematic representation of the role of IL-33 and miR-29a in tendon pathology. Tendon injuries or repetitive micro tears causing stress of tendon cells result in the release of IL-33 from tenocytes or immune cells and the downstream phosphorylation of NFκB which in turn repressesmiR-29acausing an increase in collagen type 3 and sST2 production. IL-33 may also increase collagen synthesis in an ERK-dependent manner. The increased presence of collagen 3 reduces the tendon tensile strength lending to early tendon failure. However, elevated sST2 may act, in a feedback loop fashion, as a protective mechanism by removing excess IL-33 from the system. Figure 6: Schematic representation of the role of IL-33 and miR-29a in tendon pathology. Tendon injuries or repetitive micro tears causing stress of tendon cells result in the release of IL-33 from tenocytes or immune cells and the downstream phosphorylation of NFκB which in turn represses miR-29a causing an increase in collagen type 3 and sST2 production. IL-33 may also increase collagen synthesis in an ERK-dependent manner. The increased presence of collagen 3 reduces the tendon tensile strength lending to early tendon failure. However, elevated sST2 may act, in a feedback loop fashion, as a protective mechanism by removing excess IL-33 from the system. Full size image On the basis of this work, we propose IL-33 as an influential alarmin in the unmet clinical area of early tendon injury and tendinopathy, which may be important in the balance between reparation and degeneration. A previously unrecognized role for miR-29a as a post-transcriptional regulator of matrix/inflammatory genes in tendon healing and tendinopathy has been uncovered. One of the great promises of exploiting miRNAs for therapeutic purposes has been the potential of a single miRNA to regulate functionally convergent target genes. Our discovery of a single miRNA-dependent regulatory pathway in early tissue healing highlights miR-29a replacement therapy as a promising therapeutic option for tendinopathy with implications for other human pathologies in which matrix dysregulation is implicated. Human model of tendinopathy All procedures and protocols were approved by the Ethics Committee under ACEC No. 99/101 with informed consent obtained as per standard operative procedures. Seventeen supraspinatus tendon (torn tendon representing established pathology) samples (sample size based on our previous findings of significance with 10–12 patient samples [46] , [47] ) were collected from patients with rotator cuff tears undergoing shoulder surgery ( Supplementary Table 1 ). The mean age of the rotator cuff ruptured patients was 54 years (range, 35–70 years)—the mean tear size was 2.5 cm. Samples of the subscapularis tendon (representing ‘early pathology’) were also collected from the same patients. Patients were only included if there was no clinically detectable evidence of subscapularis tendinopathy on a preoperative MRI scan or macroscopic damage to the subscapularis tendon at the time of arthroscopy—by these criteria, they represented a truly preclinical cohort. An independent control group was obtained comprising 10 samples of subscapularis tendon collected from patients undergoing arthroscopic surgery for shoulder stabilization without rotator cuff tears. The absence of rotator cuff tears was confirmed by arthroscopic examination. The mean age of the control group was 35 years (range, 20–41 years). All torn supraspinatus samples showed Grade 4 changes consistent with marked degeneration, mucoid change and frank chondroid metaplasia. Matched subscapularis tendon showed Grade 2–3 changes indicative of moderate-advanced tendinopathy. All control samples were classified as Grade 1 consistent with normal fibrotendinous tissue with large distinct collagen fibrils. There were no significant correlations between Bonar score and the mean duration of symptoms or age of the patient cohort. Tissue collection and preparation Arthroscopic repair of the rotator cuff was carried out using the standard three-portal technique and the cross-sectional size of the rotator cuff tear was estimated and recorded as described previously [48] . The subscapularis tendon was harvested arthroscopically from the superior border of the tendon 1 cm lateral to the glenoid labrum. The supraspinatus tendon was harvested from within 1.5 cm of the edge of the tear before surgical repair. For immunohistochemical staining, the tissue samples were immediately fixed in 10% (v/v) formalin for 4 to 6 h and then embedded in paraffin. Sections were cut to 5 μm thickness using a Leica-LM microtome (Leica Microsystems, Germany) and placed onto Superfrost Ultra Plus glass slides (Gerhard Menzel, Germany). Paraffin was then removed from the tissue sections with xylene, rehydrated in graded alcohol and used for histological and immunohistochemical staining according to previously established methodologies [49] . Human tendon-derived cells were explanted from hamstring tendon tissue of five patients (aged 18–30 years) undergoing hamstring tendon anterior cruciate ligament reconstruction. Normal tendinous structure and Bonar scoring was ensured by histology before inclusion. Cultures were maintained at 37 °C in a humidified atmosphere of 5% CO 2 for 28 days. Cells were subcultured and trypsinized at subconfluency. Cells from the third and fourth passage were used and tenocyte lineage was confirmed by tenascin C, CD55 and scleraxis staining as per our previous protocols [46] . We recognize the limitations of anatomical, environmental and biomechanical differences between rotator cuff and hamstring tendons. However, our rationale behind using these models is based on our previous reports utiliszng the same systems [23] , [46] and ultimately, within the field, they remain the ‘gold standard ‘ for allowing comparative molecular investigation of the early events in tendon injury/disease [50] . Histology and immunohistochemistry Human tendon sections were stained with haematoxylin and eosin and toluidine blue for determination of the degree of tendinopathy as assessed by a modified version of the Bonar score [51] (Grade 4, marked tendinopathy; 3, advanced tendinopathy; 2, moderate degeneration; 1, mild degeneration; 0, normal tendon). This included the presence or absence of oedema and degeneration together with the degree of fibroblast cellularity and chondroid metaplasia. Thereafter, the sections were stained with antibodies directed against the following markers:—IL-33 (Alexis ALX-804–840, mouse monoclonal 5 μg ml −1 ), ST2 (R&D Systems, Europe, Clone 97203, mouse monoclonal 15 μg ml −1 ), IL-1RaCP (ProSci 2131, rabbit polyclonal 5 μg ml −1 ), CD68 (pan macrophages, clone KP-1, Vector 1 μg ml −1 ), CD3 (T cells, cone LN10, Vector Labs 1.25 μg ml −1 ), CD4 (T helper cells clone 1F6, Dako Labs 1 μg ml −1 ), CD206 (M2 macrophages, R&D Systems, AF2534 5 μg ml −1 ) and mast cell tryptase (Mast cells clone 10D11, Vector Labs 1 μg ml −1 ). Endogenous peroxidase activity was quenched with 3% (v/v) H 2 O 2 , and nonspecific antibody binding blocked with 2.5% horse serum in TBST (Tris-buffered saline with Tween 20) buffer for 30 min. Antigen retrieval was performed in 0.01 M citrate buffer for 20 min in a microwave. Sections were incubated with primary antibody in 2.5% (w/v) horse serum/human serum/TBST at 4 °C overnight. After two washes, the slides were incubated with Vector ImmPRESS Reagent kit as per the manufacturer’s instructions for 30 min. The slides were washed and incubated with Vector ImmPACT DAB chromagen solution for 2 min, followed by extensive washing. Finally, the sections were counterstained with haematoxylin. Positive (human tonsil tissue) specimens were included, in addition to the surgical specimens for each individual antibody staining technique. Omission of primary antibody and use of negative control isotype confirmed the specificity of staining. We applied a scoring system based on previous methods [47] to quantify the immunohistochemical staining. Ten random high power fields ( × 400) were evaluated by three independent assessors (N.L.M., J.H.R., A.L.C.). In each field, the number of positive and negatively stained cells were counted and the percentage of positive cells calculated giving the following semi-quantitative grading; Grade 0, no staining; Grade 1, <10% cells stained positive; 2, 10–20% cells stained positive; Grade 3, >20% cells positive. Mouse tendon sections were processed using the above protocol with antibodies directed against the following markers:—IL-33 (R&D systems AF3626, mouse monoclonal), ST2 (R&D Systems Clone 97203, mouse monoclonal 15 μg ml −1 ) and F4/80 (Serotec clone CI:A3-1, mouse monoclonal 20 μg ml −1 )). Matrix regulation Total soluble collagen was measured from cell culture supernatants using the Sircol assay kit (Biocolor, Carrickfergus, Northern Ireland) according to the manufacturer’s protocol. Sircol dye reagent (1 ml) was added to test sample (100 μl) and mixed for 30 min at room temperature. The collagen–dye complex was precipitated by centrifugation at 10,000 g for 10 min and then washed twice with 500 μl of ethanol. The pellet was dissolved in 500 μl of alkali reagent. Absorbance was measured by microplate reader at 540 nm, with standard provided by the manufacturer. The concentrations of human and mouse collagen 1 and 3 were assessed using ELISA (USCNK Life Science Inc) with colour change measured at 450 nm by microplate reader, along with standards supplier by the manufacturer. Signalling experiments Phosphorylation status of MAPKs (mitogen-activated protein kinases), extracellular signal regulated kinases (ERK1/2), c-Jun N-terminal kinases (JNKs) and p38 isoforms were evaluated using the Human Phospho-MAPK Array (R&D Systems) as per the manufacturer’s instructions. The ERK inhibitor (FR180204) was purchased from CalbioChem (Merck KGaA, Germany) and used at IC 50 =10 μM, a concentration previously determined to offer optimal specific inhibition relative to off target effects, which was used previously in our laboratory [52] . Phosphorylation of NF-κB p65 was assessed using the InstantOne ELISA in cell lysates from treated and untreated tenocytes. Absorbance was measured at 450 nm by microplate reader with positive and negative controls supplied by the manufacturer. The relative absorbance of stimulated versus unstimulated cells was used to assess the total or phosphorylated NF-κB p65 in each sample. The NF-κB inhibitor (SN50) was purchased from CalbioChem (Merck KGaA, Germany) and used at IC 50 =11 nM. RNA extraction and quantitative PCR The cells isolated from experiments were placed in Trizol before mRNA extraction. QIAgen mini columns (Qiagen) were used for the RNA clean-up with an incorporated on column DNAse step as per the manufacturer’s instructions. cDNA was prepared from RNA samples according to AffinityScript (Agilent Technologies) multiple temperature cDNA synthesis kit as per the manufacturer’s instructions. Real-time PCR was performed using SYBR green or Taqman FastMix (Applied Biosystems,) according to whether a probe was used with the primers. The cDNA was diluted 1 in 5 using RNase-free water. Each sample was analysed in triplicate. Primers (Integrated DNA Technologies, Belgium) were as follows: human GAPDH , 5′-TCG ACA GTC AGC CGC ATC TTC TTT-3′ (f) and 5′-ACC AAA TCC GTT GAC TCC GAC CTT-3′ (r); mouse Gapdh 5′-TGG CAA AGT GGA GAT TGT TGC C-3′ (f) and 5′-AAG ATG GTG ATG GGC TTC CCG-3′ (r); human 18S , 5′-GTA ACC CGT TGA ACC CCA TT-3′ (f) and 5′-CCA TCC AAT CGG TAG TAG CG -3′ (r); mouse 18s , 5′-TTG ACG GAA GGG CAC CAC CAG-3′ (f) and 5′-CTC CTT AAT GTC ACG CAC GAT TTC-3′ (r); human U6 , 5′-GTG CTC GCT TCG GCA GCA CAT ATA C-3′ (f) and 5′-AAA AAT ATG GAA CGC TTC ACG AAT TTG-3′ (r); human IL33 , 5′-GGA AGA ACA CAG CAA GCA AAG CCT-3′ (f) and 5′-TAA GGC CAG AGC GGA GCT TCA TAA-3′ (r); murine Il33 , 5′-GGA AGA ACA CAG CAA GCA AAG CCT-3′ (f) and 5′-TAA GGC CAG AGC GGA GCT TCA TAA-3′ (r); total human ST2 , 5′-ACA ACT GGA CAG CAC CTC TTG AGT-3′ (f) and 5′-ACC TGC GTC CTC AGT CAT CAC ATT-3′ (r); murine sSt2 , 5′-CCA ATG TCC CTT GTA GTC GG (f) and CTT GTT CTC CCC GCA GTC (r), TCC CCA TCT CCT CAC CTC CCT TAA T-3′ (probe); mouse mSt2 , 5′-TCT GCT ATT CTG GAT ACT GCT TTC-3′ (f) and 5′-TCT GTG GAG TAC TTT GTT CAC C-3′ (r), 5′-AGA GAC CTG TTA CCT GGG CAA GAT G-3′ (probe); human mST2 , 5′-ACA AAG TGC TCT ACA CGA CTG-3′ (f) and 5′-TGT TCT GGA TTG AGG CCA C-3′ (r); 5′-CCC CAT CTG TAC TGG ATT TGT AGT TCC G-3′ (probe); human sST2 , 5′-GAG ACC TGC CAC GAT TAC AC-3′ (f) and 5′-TGT TAA ACC CTG AGT TCC CAC-3′ (r), 5′-CCC CAC ACC CCT ATC CTT TCT CCT-3′ (probe); human COL3A , 5′-TTG GCA GCA ACG ACA CAG AAA CTG-3′ (f) and 5′-TTG AGT GCA GGG TCA GCA CTA CTT-3′ (r); mouse Col3a , 5′-GCT TTG TGC AAA GTG GAA CCT GG-3′ (f) and 5′-CAA GGT GGC TGC ATC CCA ATT CAT-3′ (r); human COL1A1 , 5′-CCA TGC TGC CCT TTC TGC TCC TTT-3′ (f) and 5′-CAC TTG GGT GTT TGA GCA TTG CCT-3′ (r); mouse Col 1a1 , 5′-TTC TCC TGG CAA AGA CGG ACT CAA-3′ (f) and 5′-GGA AGC TGA AGT CAT AAC CGC CA-3′ (r). All mRNA and miRNA data sets (except Fig. 4a ) represent fold change in gene expression compared with designated control utilizing housekeeping genes GAPDH , 18S or U6 as detailed in Figure legend. Figure 4a shows threshold cycle ( C t) data for miR-29a/b/c expression in human tenocytes and human tendon tissue samples. Lower C t value represents higher message abundance. RNA isolation and quantitative PCR of miRNA Total RNA was isolated by miRNeasy kit (Qiagen). miScript Reverse Transcription Kit (Qiagen) was used for cDNA preparation. TaqMan mRNA assays (Applied Biosystems) or miScript primer assay (Qiagen) were used for quantitative determination of the expression of human miR-29a (MS00001701) miR-29b (MS00006566) and miR-29c (MS00009303) and mouse miR-29a (MS00003262), miR-29b (MS00005936) and miR-29c (MS00001379). Expressions of U6B small nuclear RNA or β-actin were used as endogenous controls. Quantification of alternative polyadenylated collagen transcripts The absolute levels of long and short 3′UTR forms of type I and III transcripts were determined by qPCR relative to standards. cDNA was generated using AffinityScript (Agilent) with both random hexamer and oligo-dT primers. SYBR green qPCR was performed using the following primers: Samples were normalized to GAPDH endogenous control. COL1A2_S FW 5′-GCCTGCCCTTCCTTGATATT-3′ COL1A2_S REV 5′-TGAAACAGACTGGGCCAATG-3′ COL1A2_L FW 5′-TCAGATACTTGAAGAATGTTGATGG-3′ COL1A2_L REV 5′-CACCACACGATACAACTCAATAC-3′ COL1A1_S FW 5′-CTTCACCTACAGCGTCACT-3′ COL1A1_S REV 5′-TTGTATTCAATCACTGTCTTGCC-3′ COL1A1_L FW 5′-CCACGACAAAGCAGAAACATC-3′ COL1A1_L REV 5′-GCAACACAGTTACACAAGGAAC-3′ COL3A1_S FW 5′-CTATGACATTGGTGGTCCTGAT-3′ COL3A1_S REV 5′-TGGGATTTCAGATAGAGTTTGGT-3′ COL3A1_L FW 5′-CCACCAAATACAATTCAAATGC-3′ COL3A1_L REV 5′-GATGGGCTAGGATTCAAAGA-3′ 3′RACE 3′RACE was performed on RNA that had been reverse transcribed using AffinityScript (Agilent) by sequence tagged oligo-dT primers (QT, Q0 Q1). 3′ sequences were then amplified using nest-PCR approach with gene-specific primers (GSP 1/2). Amplified products were cloned into pCR2.1TOPO (Invitrogen) and sequenced. QT 5′-CCAGTGAGCAGAGTGACGAGGACTCGAGCTCAAGCTTTTTTTTTTTTTTTTT-3′ Q0 5′-CCAGTGAGCAGAGTGACG-3′ Q1 5′-GAGGACTCGAGCTCAAGC-3′ COL1A1 GSP1 5′-CTTCCTGTAAACTCCCTCCATC-3′ COL1A1 GSP2 5′-AACAGACAAGCAACCCAAAC-3′ COL1A2 GSP1 5′-CAGACAAGCAACCCAAACTG-3′ COL1A2 GSP2 5′-AATGGGAGACAATTTCACATGG-3′ COL3A1 GSP1 5′-GCCTGCCCTTCCTTGATATT-3′ COL3A1 GSP2 5′-CCTTCCATTTCTTCTGCACATC-3′ miRNA transfection Cells (primary tenocytes) were transfected with synthetic mature miRNA for miR-29a and b or with negative control ( C. elegans miR-67 mimic labelled with Dy547, Thermo Scientific Inc.) at a final concentration of 20 nM with the use of Dharmacon DharmaFECT 3 siRNA transfection reagents (Thermo Scientific Inc.). At 48 h after transfection, the cellular lysates were collected to analyse the expression of genes of interest. Transfection efficiency (80%) was assessed by flow cytometry using the labelled Dy547 mimic ( Supplementary Fig. 7g ) and confirmed by qPCR of control-scrambled mimic and the respective miR29 family mimic. Luciferase reporter assay for targeting collagen 1 and 3 and soluble ST2 The human 2 miRNA target site was generated by annealing the oligos: for COL 1 and 3 and soluble ST2 3′UTRs that were cloned in both sense and antisense orientations downstream of the luciferase gene in pMIR-REPORT luciferase vector (Ambion). These constructs were sequenced to confirm inserts and named pMIR- COL I/COL III/ sST2 - miR29a/b/c and pMIR(A/S)- COL I/COL III/ sST2 - miR29a/b/c , and used for transfection of HEK293 cells (HEK293 cells tested negative for mycoplasma before use). HEK293 cells were cultured in 96-well plates and transfected with 0.1 μg of either pMIR- COL I/COL III/ sST2 -miR29a/b/c, pMIR(A/S)- COL I/COL III/ sST2 -miR29a/b/c or pMIR-REPORT, together with 0.01 μg of pRL-TK vector (Promega) containing Renilla luciferase and 40 nM of miR-29a or scrambled miRNA (Thermo Scientific Dharmacon). Transfections were performed using Effectene (Qiagen) according to the manufacturer’s instructions. Luciferase activity was measured 24 h after transfection using the Dual-Luciferase Reporter Assay (Promega). The 3′UTR of human sST2 was amplified from genomic DNA using the following primers (f) 5′-AGTTTAAACTGGCTTGAGAAGGCACACCGT-3′ and (r) 5′-AGTCGACGGGCCAAGAAAGGCTCCCTGG-3′, which created PmeI and SalI sites, respectively. These sites where used to clone the PCR-amplified product into the same sites of pmiRGLO (Promega). The seed regions of the two Targetscan predicted miR-29a MRE sites: 29-1 and 29-2 were mutated using the QuickChange site-directed mutagenesis kit (Agilent). Each vector along with miR-29a or scrambled control mimic were transfected into HEK293 cells using Attactene (Qiagen) according to the manufacturer’s instructions. Luciferase activity was measured 24 h later using Dual-Glo luciferase assay (Promega) with luciferase activity being normalized to Renilla. Normalized luciferase activity was expressed as a percentage of scrambled control for the same constructs. Cytokine production Cytokine concentration in the supernatant of cultured human tenocytes was determined by 25-Plex human cytokine assay (with 25 separate human cytokines) using Luminex (Luminex Corp). Animals and patellar tendon injury model BALB/c mice were purchased from Charles River. St2 −/− mice (of BALB/c background) were originally provided by Dr Andrew McKenzie (LMB, Cambridge). Mice were maintained at the Central Research Facility, University of Glasgow. All animal experimentation and husbandry were according to the UK Government Home Office Project License. All protocols were approved by the Glasgow University local Ethical Review Panel. Mice were used at 10–12 weeks old and were age matched for each independent experiment. In vivo experimental protocols are depicted in Supplementary Fig. 7e,f,h ). In preparation for the surgical procedure, mice were anaesthetized with a mixture of isofluorane (3%) and oxygen (1%) and both hind limbs were shaved. During surgical procedures, anaesthesia was delivered via a nose cone with the level of isofluorane reduced to 1% with oxygen. Following a skin incision, two cuts parallel to the tendon were made in the retinaculum on each side, a set of flat faced scissors were then placed underneath the patellar tendon. With the scissor blades serving as a support, a 0.75-mm diameter biopsy punch (World Precision Instruments) was used to create a full thickness partial transection in the right patellar tendon. The left patellar tendon underwent a sham procedure, which consisted of only placing the plastic backing underneath the tendon without creating and injury. The skin wounds were closed with skin staples and the mice were killed at day 1, 3, 7 or 21 post surgery. Mice were killed by CO 2 inhalation and immediately weighted. Each group contained 16 mice ( n =8, St2 −/− and 8 WT) per time point. These experiments were repeated on four separate occasions. To test if IL-33 induced tendon matrix dysregulation, a cytokine injection model was used. IL-33 was tested in a previously reported model initially described for the application of IL-23 or IL-22 (refs 53 , 54 ). St2 −/− mice ( n =4 per group/treatment/experiment) were injected intraperitoneally daily with IL-33 (0.4 μg per mouse diluted in 100 μl PBS) on days − 3, − 2, − 1 and the day of injury (day 0). Mice were culled 24 h after the final injection as per protocol. Control mice similarly received an equal volume of PBS. We also tested neutralizing antibodies to IL-33 (0.5 μg ml −1 , R&D systems) by injecting (i.p) the antibody or normal IgG control immediately post injury in WT and St2 −/− mice (four per group/treatment/experiment). miR-29a mimic (50 ng ml −1 in 0.1 ml) was delivered via direct injection to injured (immediately post injury) and uninjured mice tendons ( n =6 per group/treatment/experiment). Control mice similarly received an equal volume of PBS. During these procedures, the GCP principles were applied. All samples were labelled in a numerical fashion and were then blinded during all further experimental methodology. Numerical codes were only revealed post experiment and analysis. Biomechanical analysis For biomechanical analysis, the patellar tendons of mice from each group were injured and eight mice killed at one of the four time points for mechanical testing as described previously by Lin et al. [10] ( Supplementary Fig. 7f ). On the basis of previous experiments, a sample size of eight per group offered 95% confidence interval that a 50% difference between injured and control littermate animals would be detected. In brief, the patellar tendons were dissected and cleaned, leaving only the patella, patellar tendon and tibia as one unit. Tendon width and thickness were then quantified and cross-sectional area was calculated as the product of the two. The tibia was then embedded in Isopon p38 (High Build Cellulose Filler) in a custom-designed fixture and secured in place in a metal clamp. The patella was held in place by vice grips used with the BOSE ElectroForce 3200 test instrument. Each tendon specimen underwent the following protocol immersed in a 37 °C saline bath—reloaded to 0.02 N, preconditioned for 10 cycles from 0.02 to 0.04 at a rate of 0.1% s −1 (0.003 mm s −1 ), and held for 10 s. Immediately, a stress relaxation experiment was performed by elongating the tendon to a strain of 5% (0.15 mm) at a rate of 25% (0.75 mm/s), followed by a relaxation for 600 s. Finally, a ramp to failure was applied at a rate of 0.1% s −1 (0.003 mm s −1 ). From these tests, maximum stress was determined and modulus was calculated using linear regression from the near linear region of the stress strain curve. Statistical analysis All results are shown as mean±s.d. and all statistical analysis was performed using Student’s t -test, ANOVA (analysis of variance) test or Mann–Whitney test U -test, as indicated in figure legends, using the Graph Pad Prism 5 software. A P value of <0.05 was considered statistically significant. How to cite this article: Millar, N. L. et al. MicroRNA29a regulates IL-33-mediated tissue remodelling in tendon disease. Nat. Commun. 6:6774 doi: 10.1038/ncomms7774 (2015).